Nonreciprocal plasmonics enables giant enhancement of thin-film Faraday rotation Light propagation is usually reciprocal. However, a static magnetic field along the propagation direction can break the time-reversal symmetry in the presence of magneto-optical materials. The Faraday effect in magneto-optical materials rotates the polarization plane of light, and when light travels backward the polarization is further rotated. This is applied in optical isolators, which are of crucial importance in optical systems. Faraday isolators are typically bulky due to the weak Faraday effect of available magneto-optical materials. The growing research endeavour in integrated optics demands thin-film Faraday rotators and enhancement of the Faraday effect. Here, we report significant enhancement of Faraday rotation by hybridizing plasmonics with magneto-optics. By fabricating plasmonic nanostructures on laser-deposited magneto-optical thin films, Faraday rotation is enhanced by one order of magnitude in our experiment, while high transparency is maintained. We elucidate the enhanced Faraday effect by the interplay between plasmons and different photonic waveguide modes in our system. Plasmonics provides abundant routes to manipulate light–matter interaction by nanostructures that can localize light and alter the field distribution at sub-wavelength scale [1] . Combining plasmonics with magneto-optics is of particular interest [2] , [3] , [4] , [5] , [6] , [7] , [8] , as it enables sophisticated control of magneto-optical material properties, which can lead to many optical devices where magnetism is applied. For example, by hybridizing ferromagnetic and noble metal materials, the magneto-optical polar Kerr effect was enhanced, which was termed ‘magneto-plasmonics’ [9] , [10] . In this realm, Temnov et al . [11] , [12] reported plasmon interferometers, which utilized propagating surface plasmons controlled by a static magnetic field due to an adjacent ferromagnetic layer. Meanwhile, one-way waveguiding [13] and one-way extraordinary optical transmission [14] were proposed by integrating magnetic materials with a photonic crystal and spoof surface plasmons, respectively. Among the various magneto-optical effects, Faraday rotation is of special interest, as it is the key technology in optical isolation [15] , [16] . Previously, plasmonic heterostructures [17] and planar photonic crystals [18] were proposed theoretically to enhance the nonreciprocal Faraday effect, but have not yet been realized. In this work, we experimentally demonstrate large enhancement of the Faraday effect over a rather broad bandwidth. It is achieved by incorporating nonreciprocal magneto-optical material with plasmonic photonic crystal [19] , [20] , [21] . Specifically, we fabricate plasmonic nanowire arrays on magneto-optical thin films and characterize the Faraday rotation by polarimetry. Faraday rotation is increased by up to 8.9 times compared with the bare film, while high transparency is maintained. We simulate the hybrid system by numerical tools and find good agreement between simulation and experiment. Our results reveal the mechanism behind the enhancement of Faraday effect in analogy to the classical coupled oscillator model, which can be used to engineer the properties of the nonreciprocal plasmonic system. We expect our concept to find applications in nonreciprocal thin-film optical devices. Magneto-plasmonic photonic crystal We utilize periodic gold nanowires structured on a thin layer of magneto-optical material, which is deposited on a glass substrate, as depicted in Fig. 1a . Such a system allows simultaneous oscillation of plasmons and photons. A localized plasmon resonance is excited by incoming light polarized perpendicular to the wires, defined as TM-polarized incident light. (TE and TM polarizations are specified in Fig. 1 .) Besides the plasmon resonance, the nanowires introduce periodicity to the hybrid structure and hence enable light to couple into the magneto-optical thin film, which acts as a planar photonic crystal waveguide for photons [20] , [21] . The localized plasmon resonance and the waveguide resonance interact strongly, and this interaction can be tailored to engineer the magneto-optical properties. 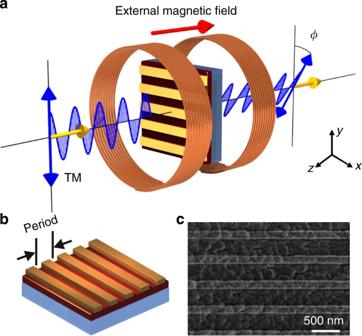Figure 1: Magneto-plasmonic photonic crystal. (a) Faraday rotation by a magneto-plasmonic photonic crystal for TM-polarized incident light, whereφis the Faraday rotation angle. At normal incidence, TM-polarized light has the electric field perpendicular to the gold wires, and TE-polarized light has the electric field parallel to the wires. (b) Schematic of the magneto-optical photonic crystal, where BIG film (dark red) is deposited on glass substrate (blue) and periodic gold nanowires (golden) are sitting atop. (c) A scanning electron microscopy image of one sample. Figure 1: Magneto-plasmonic photonic crystal. ( a ) Faraday rotation by a magneto-plasmonic photonic crystal for TM-polarized incident light, where φ is the Faraday rotation angle. At normal incidence, TM-polarized light has the electric field perpendicular to the gold wires, and TE-polarized light has the electric field parallel to the wires. ( b ) Schematic of the magneto-optical photonic crystal, where BIG film (dark red) is deposited on glass substrate (blue) and periodic gold nanowires (golden) are sitting atop. ( c ) A scanning electron microscopy image of one sample. Full size image Fabrication and characterization Three samples of plasmonic photonic crystals were fabricated, each of which consists of 120-nm wide and 65-nm thick periodic nanowires structured on top of a 150-nm thick bismuth iron garnet (BIG) thin film ( Fig. 1b ). The three samples have different periods of the nanowires, being 400, 450 and 495 nm, respectively. Figure 1c shows a scanning electron micrograph of one sample. A magnetic field of 140 mT was applied normal to the BIG film, and Faraday rotation φ of the samples was measured at normal incidence using a rotating analyser polarimeter. For TM-polarized incident light, Faraday rotation of the plasmonic photonic crystals compared with Faraday rotation of the reference BIG film is shown in Fig. 2a . 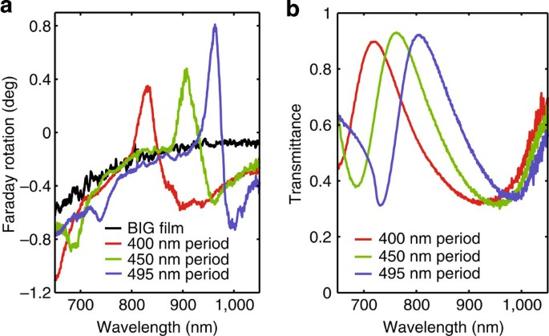Figure 2: Measured Faraday rotation and transmittance. (a) Measured Faraday rotation of the three samples at normal incidence (TM polarization), compared with measured Faraday rotation of the bare BIG film. (b) Measured transmittance of the three samples at normal incidence (TM polarization). Figure 2: Measured Faraday rotation and transmittance. ( a ) Measured Faraday rotation of the three samples at normal incidence (TM polarization), compared with measured Faraday rotation of the bare BIG film. ( b ) Measured transmittance of the three samples at normal incidence (TM polarization). Full size image The spectra of Faraday rotation display a resonant feature. As the period increases, the resonance shifts to longer wavelength and the maximum Faraday rotation increases. The sample of 495 nm period reaches a maximum Faraday rotation of 0.80° at λ =963 nm, which is 8.9 times enhancement of the −0.09° Faraday rotation of the BIG film without gold wires. The 0.80° Faraday rotation has a half-value bandwidth of 22 nm. As high transparency is favourable for the potential application of Faraday rotators, spectra of transmittance were measured for all the samples ( Fig. 2b ). The 495-nm period sample shows 36% transmittance at λ =963 nm. In comparison, the sample of 450 nm period exhibits Faraday rotation of 0.45° at λ =907 nm. Compared with −0.11° Faraday rotation of the bare BIG film, it is an enhancement of 4.1 times. The sample of 400 nm period shows Faraday rotation of 0.33° at the resonant peak of λ =831 nm. Compared with Faraday rotation of the bare BIG film, −0.17 °, there is 1.9 times enhancement. The resonant shape of the Faraday rotation spectra and transmittance spectra is directly related to the waveguide–plasmon polaritons [20] , [21] . Cross-coupling of the TM and TE modes accounts for the enhancement of Faraday rotation. Two orthogonal coupled oscillators model The responsible coupling of the TM and TE modes can be described by two orthogonal harmonic oscillators bound together by an elastic spring [22] ( Fig. 3a ). If an oscillator is excited in one direction, the oscillation is transferred to the other oscillator via the elastic spring, and thus causes reradiation of waves in the orthogonal direction. In the magneto-plasmonic photonic crystal, TM-polarized incident light induces a TM waveguide–plasmon hybrid mode, with the electric field in the BIG film oscillating in the plane perpendicular to the wires and the magnetic field oscillating along the wires [20] . 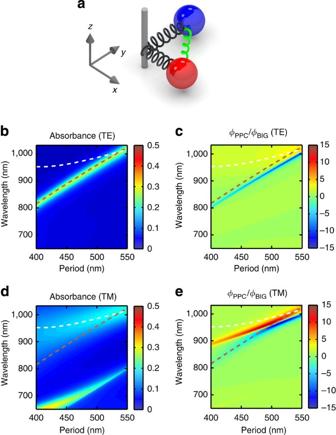Figure 3: Two orthogonal oscillators model and diagrams of absorbance and enhancement of Faraday rotation. (a) Two orthogonal harmonic oscillators bound together by an elastic spring. (b,c), Simulated diagrams of absorbance (b) and enhancement of Faraday rotationφPPC/φBIG(c) for TE-polarized incident light. (d,e) Simulated diagrams of absorbance (d) and enhancement of Faraday rotationφPPC/φBIG(e) for TM-polarized incident light. The white dashed line indicates the fundamental TM waveguide–plasmon hybrid mode and the red dashed line indicates the fundamental TE waveguide mode. In the presence of static magnetization, the permittivity of BIG can be described by a tensor [23] Figure 3: Two orthogonal oscillators model and diagrams of absorbance and enhancement of Faraday rotation. ( a ) Two orthogonal harmonic oscillators bound together by an elastic spring. ( b,c ), Simulated diagrams of absorbance ( b ) and enhancement of Faraday rotation φ PPC / φ BIG ( c ) for TE-polarized incident light. ( d,e ) Simulated diagrams of absorbance ( d ) and enhancement of Faraday rotation φ PPC / φ BIG ( e ) for TM-polarized incident light. The white dashed line indicates the fundamental TM waveguide–plasmon hybrid mode and the red dashed line indicates the fundamental TE waveguide mode. Full size image where g in the off-diagonal elements describes the magnetization-induced gyration of the material. The off-diagonal elements have a similar role as the the elastic spring in the two orthogonal oscillators model, and give rise to an additional electric field component orthogonal to the electric field of the incident light. This secondary component of the electric field oscillates and emits TE-polarized light. Consequently, the optical far-field signal acquires a TE-polarized component and the plane of polarization is rotated. Large enhancement of Faraday rotation requires strong coupling between the TE and TM modes, which is most efficient when the two modes are spectrally close and therefore can be excited simultaneously. This intuitive model is supported by numerical modelling of the plasmonic photonic crystal. Figure 3b–e shows the simulated diagrams of absorbance and the enhancement of Faraday rotation for TE- and TM-polarized incident light in dependence of the wavelength of the incident light and the period of the nanowires. The white and red dashed lines in Fig. 3b–e indicate the excitation of the fundamental TM waveguide–plasmon mode and the fundamental TE waveguide mode, respectively. In the vicinity of the intersection between the white and red lines, the TM and TE modes are excited simultaneously. As a result, the enhancement of Faraday rotation φ PPC / φ BIG for TM- and TE-polarized incident light reaches its maximum in this region as shown in Fig. 3c (here φ PPC denotes Faraday rotation of the plasmonic photonic crystals, and φ BIG denotes that of the reference BIG film). This is attributed to the effective coupling between the TM and TE modes, which can be understood via the two orthogonal oscillators model. The sample with 495 nm period has the TM and TE modes spectrally closer than the others, which leads to its highest enhancement of Faraday rotation among the samples. As the period decreases to 400 nm, the modes indicated by the white and red lines in Fig. 3b–e drift away from each other, so that the coupling between TE and TM modes becomes weaker, and the enhancement factor of Faraday rotation attenuates accordingly. Note that the maximum Faraday rotation does not coincide exactly with the crossing of the TE and TM modes. That is because, apart from the cross-coupling of the TM and TE modes and the effective generation of the secondary electric field component, Faraday rotation is also dependent on the far-field radiation of the primary electric field component. Simulation and intuitive picture of enhanced Faraday effect Simulated field distributions for the sample of 495 nm period and incident wavelength of 963 nm are depicted in Fig. 4a . The cross section of the planar photonic crystal is illustrated by white solid lines, with the rectangles representing the gold wires structured on the BIG film. The field distributions clearly reveal that a TM waveguide–plasmon hybrid mode and a TE waveguide mode are indeed excited simultaneously. The excitation of the TM and TE modes can be understood in the following way. For incident light with TE polarization, the electric field is polarized along the wires. When the TE waveguide mode is excited, light is diffracted into the BIG film by the periodic nanowires with non-zero diffraction orders, so that it experiences total internal reflection at the boundaries of the waveguiding slab and bounces back and forth inside the slab. As a result, the electric field is enhanced in the BIG film and forms the pattern as shown in Fig. 4a . For incident light with TM polarization, instead of the electric field, the magnetic field is polarized along the wires and concentrated in the waveguide at the resonance of the TM mode ( Fig. 4b ), but showing a slightly different field distribution pattern compared with Fig. 4a . The difference is introduced by the plasmon resonance excited only for TM-polarized incident light, which hybridizes with the waveguide resonance. When the TE or TM modes are excited, light travels up and down inside the slab, and each time a small amount of Faraday rotation takes place, which accumulates to enhance Faraday rotation of the light that couples out (as depicted in Fig. 4c ). Thus, we observe the enhanced Faraday rotation as demonstrated before in the diagrams of Fig. 3c . 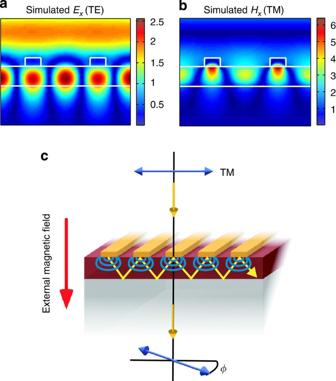Figure 4: Simulated field distribution and mechanism of the enhanced Faraday rotation. (a,b) Simulated spatial distribution of |Ex| at TE-polarized incident light (a) and |Hx| at TM-polarized incident light (b) atλ=963 nm. The amplitudes of the fields are normalized to that of the incident light. (c) Simultaneous excitation of plasmon resonance and waveguide mode for TM-polarized incident light contributes to enhanced Faraday rotationφ. Inside the BIG film, the blue lines near the gold wires indicate the field enhancement due to the plasmon resonance, and the yellow line implies light bouncing inside the slab due to the excitation of the waveguide mode. Figure 4: Simulated field distribution and mechanism of the enhanced Faraday rotation. ( a,b ) Simulated spatial distribution of | E x | at TE-polarized incident light ( a ) and | H x | at TM-polarized incident light ( b ) at λ =963 nm. The amplitudes of the fields are normalized to that of the incident light. ( c ) Simultaneous excitation of plasmon resonance and waveguide mode for TM-polarized incident light contributes to enhanced Faraday rotation φ . Inside the BIG film, the blue lines near the gold wires indicate the field enhancement due to the plasmon resonance, and the yellow line implies light bouncing inside the slab due to the excitation of the waveguide mode. 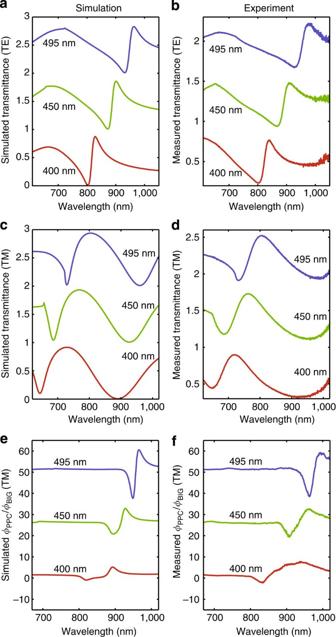Figure 5: Simulation of transmittance and enhancement of Faraday rotation compared with measurement. The spectra are shifted vertically for clarity. (a,b) Simulated transmittance for TE-polarized incident light of the three samples (a) compared with the measured transmittance (b). (c,d) Simulated transmittance for TM-polarized incident light (c) compared with the measured transmittance (d). (e,f) Simulated enhancement of Faraday rotationφPPC/φBIGfor TM-polarized incident light (e) compared with the measured enhancement (f). Full size image Transmittance and enhancement of Faraday rotation Figure 5 compares the simulated transmittance for TE- and TM-polarized incident light ( Fig. 5a ) with the measured transmittance ( Fig. 5b ). For TE polarization, a resonant waveguide mode leads to a dip in the transmittance spectra, which moves to longer wavelength when the period increases ( Fig. 5a ). It occurs at 803, 871 and 932 nm, respectively. TM-polarized incident light excites a waveguide–plasmon hybrid mode, which manifests itself by splitting of the resonance, that is, two dips in the transmittance spectra. At the transmittance dip at shorter wavelength, the waveguide resonance is dominating the mode. The resonance is therefore sharper and the corresponding wavelength increases considerably with the period. At the transmittance dip at longer wavelength, the localized plasmon resonance has a larger role, and consequently the change of the resonant wavelength is smaller (see Fig. 2b for better visualization). As the period increases, the TE waveguide mode shifts faster than the TM transmittance dip at longer wavelength, and the two move spectrally closer. The enhancement of Faraday rotation φ PPC / φ BIG , therefore, rises with increasing period, as observed in both simulation and experiment ( Fig. 5e ). The good agreement between simulation and measurement proves the numerical method as a sufficient tool to model and design the magneto-plasmonic system. Figure 5: Simulation of transmittance and enhancement of Faraday rotation compared with measurement. The spectra are shifted vertically for clarity. ( a , b ) Simulated transmittance for TE-polarized incident light of the three samples ( a ) compared with the measured transmittance ( b ). ( c , d ) Simulated transmittance for TM-polarized incident light ( c ) compared with the measured transmittance ( d ). ( e,f ) Simulated enhancement of Faraday rotation φ PPC / φ BIG for TM-polarized incident light ( e ) compared with the measured enhancement ( f ). Full size image Based on our understanding of the underlying mechanism, the enhancement of Faraday effect by hybridizing plasmonics and nonreciprocal magneto-optical materials can be modulated by the geometry of the plasmonic structures. Large enhancement of Faraday rotation can be attained by tuning the oscillations of plasmons and photons in the two orthogonal directions of the polarization plane such that they overlap spectrally. In our results, the enhancement of Faraday rotation is rather broadband due to the plasmonic nature of the system, which is beneficial for potential applications. Leveraging the coupling between the plasmonic resonance and the photonic crystal waveguide resonance may offer extra freedom to control the transparency of the system. In conclusion, we have demonstrated the largest plasmonic enhancement of Faraday rotation up to now. Our study provides insight into the dynamics of the intricate interaction among plasmons, photons and magneto-optical activity. The correlation between the optical and magneto-optical properties can be applied to other plasmon-enhanced effects, such as nonlinear harmonic generation [24] , light emitting [25] and optical chirality [26] . We expect the concept of nonreciprocal plasmonics to pave the way towards nonreciprocal thin-film optical devices that are highly integrable. Incorporating our concept with more efficient magneto-optical materials will yield larger thin-film Faraday effect demanded by potential applications. The concept may find useful applications in magnetically controlled light modulation and polarization modulation [27] , current sensing, magnetic microscopy, nonreciprocal optical antennas [28] , optical circulators [29] , and so on. It is feasible for large-area fabrication, which could be applied as nonreciprocal optical coatings, and can be integrated into optical fibre systems. The hybridization of plasmonics with magneto-optics offers the possibilities to enhance the magneto-optical effect and to engineer the working wavelength simultaneously. Fabrication and measurement The BIG film was prepared by pulsed laser deposition [30] , [31] , [32] . First, a thin buffering layer of 10-nm yttrium iron garnet (YIG, Y 3 Fe 5 O 12 ) was deposited on a glass substrate and was annealed at 1,000 °C. After that, another layer of 140 nm BIG (Bi 3 Fe 5 O 12 ) was deposited on the YIG buffering layer. As the next step, gold nanowires were fabricated on the BIG film by electron beam lithography and a subsequent lift-off process. The samples were first characterized by a white-light spectrometer at normal incidence and the result was compared with numerical simulation. They were then placed in a set of permanent ring magnets and mounted in a rotating analyser polarimeter. A white-light laser source and a high-resolution spectrometer were used in the polarimeter. A polarizer was carefully aligned to give TE and TM incident light. Faraday rotation was deduced from the angle of the rotating analyser with minimum transmission. Numerical simulation The optical properties of the magneto-plasmonic photonic crystals, such as the far-field spectra and the mode dispersion, have been modelled by the Fourier modal method with adaptive spatial resolution [33] . The permittivity tensor of BIG is slightly dispersive over the spectrum from 650 nm to 1050, nm, and the average value of the tensor with and g =0.016– i 0.0092 is adopted in the numerical simulation. The permittivity of glass is ε glass =2.13 and the dispersion of gold [34] is taken into consideration. The position of the modes overlaps approximately with the local absorbance maxima ( Fig. 3b ). They are found in the numerical simulation as poles of the scattering matrix on the complex frequency plane [33] . Faraday rotation and group velocity The large enhancement of Faraday rotation can also be associated with a vanishing group velocity v g at resonance. The relation between Faraday rotation and group velocity can be expressed as so-called specific Faraday rotation, ( [17] , [35] ), with being the TM-to-TE conversion efficiency. The TM-to-TE conversion efficiency is determined by the gyrotropic property of the magneto-optical waveguide (analogous to the elastic spring in the two coupled oscillators model). The density of states of the TM and TE modes and (analogous to the amplitude of the two harmonic oscillators in the Born–Kuhn model) are represented by the eigenfunctions of the electric field in TM and TE polarization. The expression was obtained by applying a two-coupled wave approach [35] with ω as light frequency and ‹ Q › as the magneto-optical parameter averaged along the period of the structure. Vanishing v g implies an increase of the effective length of light–matter interaction and contributes to the observed drastic enhancement of Faraday rotation. How to cite this article: Chin, J.Y. et al . Nonreciprocal plasmonics enables giant enhancement of thin-film Faraday rotation. Nat. Commun. 4:1599 doi: 10.1038/ncomms2609 (2013).